Decoupling the spread of grasslands from the evolution of grazer-type herbivores in South America The evolution of high-crowned cheek teeth (hypsodonty) in herbivorous mammals during the late Cenozoic is classically regarded as an adaptive response to the near-global spread of grass-dominated habitats. Precocious hypsodonty in middle Eocene ( ∼ 38 million years (Myr) ago) faunas from Patagonia, South America, is therefore thought to signal Earth’s first grasslands, 20 million years earlier than elsewhere. Here, using a high-resolution, 43–18 million-year record of plant silica (phytoliths) from Patagonia, we show that although open-habitat grasses existed in southern South America since the middle Eocene ( ∼ 40 Myr ago), they were minor floral components in overall forested habitats between 40 and 18 Myr ago. Thus, distinctly different, continent-specific environmental conditions (arid grasslands versus ash-laden forests) triggered convergent cheek–tooth evolution in Cenozoic herbivores. Hypsodonty evolution is an important example where the present is an insufficient key to the past, and contextual information from fossils is vital for understanding processes of adaptation. Grasslands today cover 40% of Earth’s land surface and provide habitat and food for billions of animals, including humans [1] . Since the late 19th century, researchers from T.H. Huxley to H.F. Osborn and G.G. Simpson have viewed the Cenozoic assembly of this vitally important biome as a classic example of natural selection over macroevolutionary time scales, whereby mammals evolved hypsodont teeth and large size in response to the worldwide spread of grass-dominated vegetation [2] , [3] . The significance of hypsodonty in this context is that it prolongs the life of teeth in herbivores that deal with abundant abrasives, such as silica-rich grasses and wind-blown dust, in these open, arid habitats [4] , [5] . Palaeobotanical data in the form of phytolith assemblages in central North America and western Eurasia have supported the notion of hypsodonty as an adaptive response, indicating that herbivores in these regions evolved high-crowned cheek teeth in the context of existing grasslands [6] , [7] . Consequently, the increasing cheek–tooth crown heights in nearly all large herbivore lineages in faunas from Patagonia, southern South America, starting in the middle Eocene ( ∼ 38 Myr ago) [8] ( Fig. 1 ) are viewed as marking an unexpectedly early spread of grass-dominated habitats [3] . Consistent with this pattern, sparse phytolith records from Patagonia, Argentina, have been interpreted as showing the emergence of subtropical grasslands by 40 Myr ago [9] , [10] ; similarly, accumulations of dung beetle brood balls from the middle Eocene onward are likened to those found in the African savannah today [11] . In contrast, palynofloral and plant macrofossil data from southern South America suggest that although grasses were present by the early Eocene [12] , the region was forest covered during the Eocene and Oligocene, with open and grass-dominated habitats becoming widespread only in the late Miocene [13] . 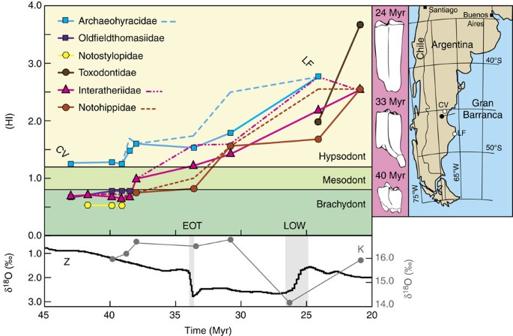Figure 1: Hypsodonty evolution in Patagonia and map of fossil localities. History of tooth crown height/width (HI) for notoungulates shows precocious hypsodonty (>30 Myr ago) in multiple families. Solid symbols, solid lines=average HI, dashed lines=maximum HI. CV=Cañadon Vaca; LF=La Flecha. Relative temperature based on benthic foraminifera δ18O (‘Z’) and local tooth enamel δ18OPO4(‘K’) for reference; EOT=Eocene-Oligocene transition; LOW=late Oligocene warming. Sketches illustrate Interatheriidae hypsodonty evolution. References inSupplementary Information. Figure 1: Hypsodonty evolution in Patagonia and map of fossil localities. History of tooth crown height/width (HI) for notoungulates shows precocious hypsodonty (>30 Myr ago) in multiple families. Solid symbols, solid lines=average HI, dashed lines=maximum HI. CV=Cañadon Vaca; LF=La Flecha. Relative temperature based on benthic foraminifera δ 18 O (‘Z’) and local tooth enamel δ 18 O PO4 (‘K’) for reference; EOT=Eocene-Oligocene transition; LOW=late Oligocene warming. Sketches illustrate Interatheriidae hypsodonty evolution. References in Supplementary Information . Full size image We tested the ‘South American early grassland’ hypothesis by developing a high-resolution temporal succession of phytolith assemblages through the Sarmiento Formation at Gran Barranca, Chubut Province, Argentina ( Figs 2 , 3 ). We analysed these assemblages following the methods of Strömberg [14] to make them directly comparable to phytolith records in North America and Eurasia [7] , [14] . Phytolith assemblage analysis provides information about vegetation type, specifically the relative abundances and types of grasses. In particular, phytoliths can distinguish preferentially forest-dwelling grasses (for example, bambusoids, basal grasses) from open-habitat grasses (members of the Pooideae and PACMAD (Panicoideae, Arundinoideae, Chloridoideae, Centothecoideae, Micrairoideae, Aristidoideae and Danthonioideae) grass sub-clades) [15] . 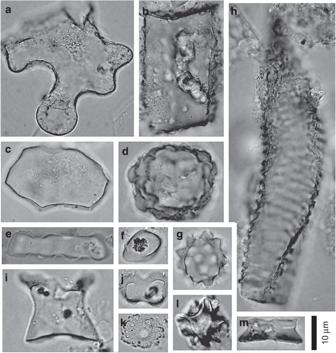Figure 2: Examples of phytoliths from the Sarmiento formation. (a) Anticlinal epidermis‡; (b) ornamented blocky body‡; (c) polyhedral epidermis‡; (d) large nodular body‡; (e) crenate (Pooideae)*,o; (f) conical rondel*,o; (g) echinate sphere (palm)‡; (h) tracheary element‡; (i) irregular, faceted/ornamented, tall bilobate (Bambusoideae?)*,‡; (j) simple bilobate (PACMAD)*,o; (k) sedge platew; (l)Costus/Canna(Zingiberales) phytolith‡; and (m) bilobate with faceted top (Danthonioideae?/Bambusoideae?)*,o. Sample numbers and further explanation of classification system used inSupplementary MethodsandSupplementary Table S5. *Grass silica short cell;‡forest indicator;oopen habitat indicator;wwetland indicator. Figure 2: Examples of phytoliths from the Sarmiento formation. ( a ) Anticlinal epidermis ‡ ; ( b ) ornamented blocky body ‡ ; ( c ) polyhedral epidermis ‡ ; ( d ) large nodular body ‡ ; ( e ) crenate (Pooideae)* ,o ; ( f ) conical rondel* ,o ; ( g ) echinate sphere (palm) ‡ ; ( h ) tracheary element ‡ ; ( i ) irregular, faceted/ornamented, tall bilobate (Bambusoideae? )* ,‡ ; ( j ) simple bilobate (PACMAD)* ,o ; ( k ) sedge plate w ; ( l ) Costus/Canna (Zingiberales) phytolith ‡ ; and ( m ) bilobate with faceted top (Danthonioideae?/Bambusoideae? )* ,o . Sample numbers and further explanation of classification system used in Supplementary Methods and Supplementary Table S5 . *Grass silica short cell; ‡ forest indicator; o open habitat indicator; w wetland indicator. 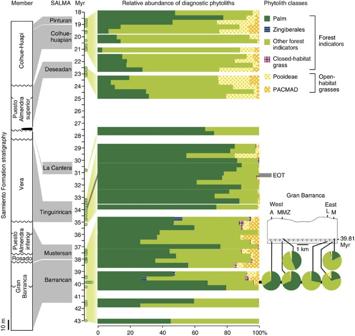Figure 3: Eocene–Miocene phytolith records from Gran Barranca and Cañadon Vaca. West–east vegetation variation at 39.81 Myr ago at Gran Barranca (profiles A, MMZ, L, M). Small green circles=age of phytolith assemblages based on a Sarmiento Formation age model; note that one sample near the base of the formation was only analysed semi-quantitatively; SALMA=South American land mammal age, EOT=Eocene–Oligocene transition. Full size image Figure 3: Eocene–Miocene phytolith records from Gran Barranca and Cañadon Vaca. West–east vegetation variation at 39.81 Myr ago at Gran Barranca (profiles A, MMZ, L, M). Small green circles=age of phytolith assemblages based on a Sarmiento Formation age model; note that one sample near the base of the formation was only analysed semi-quantitatively; SALMA=South American land mammal age, EOT=Eocene–Oligocene transition. Full size image Spanning 42–18.5 Myr ago, the Sarmiento Formation at Gran Barranca arguably holds the most complete and important record of South American faunal change, with over 80 faunal levels chronicling the shift in herbivore faunas from dominantly low-crowned to increasingly high-crowned forms [8] , [9] ( Fig. 1 ). Extensive magneto- [16] and chronostratigraphic work [17] , [18] there provides a robust temporal framework for detailed study of ecosystem change. We analysed 53 representative phytolith assemblages distributed throughout the Sarmiento Formation; five additional assemblages were analysed along the 7-km outcrop of a single prominent ash bed to investigate spatial heterogeneity in vegetation. Our data show that closed, palm-rich forests covered the region in the Eocene–Oligocene and, although open-habitat grasses became more abundant (<25%) after ∼ 23 Myr ago, habitats remained forested overall. Given the absence of grasslands, precocious hypsodonty in South America was likely not an adaptation to open, grass-dominated vegetation, but rather a response to dietary grit from abundant ash in the context of subtropical forests. Middle Eocene–Oligocene vegetation structure Diverse forest indicator (FI) phytolith morphotypes ( Fig. 2 ), including forms characteristic of palms and woody dicotyledons, dominate assemblages throughout the section ( Fig. 3 ). Notably, palms were abundant in Eocene and early Oligocene ecosystems at Gran Barranca. Grass short-cell phytoliths occur only sparsely in middle Eocene samples from near the base of the Sarmiento Formation ( ∼ 42 Myr ago) and in nearby Vacan-aged deposits ( ∼ 43 Myr ago; Fig. 1 ), indicating that grasses formed a minor part of vegetation at this time. Starting at 39.8 Myr ago, distinct short cells sharing similarities with both bambusoid grasses (for example, Chusquea ) and members of the open-habitat PACMAD clade Danthonioideae (for example, Danthonia ) become evident in grass communities. In addition, open-habitat pooid morphotypes occur rarely, as do forms typical of bambusoid or basal grasses. However, during this interval, grasses overall were rare, constituting on average only 6% of phytolith assemblages. The assemblages also contain low abundances of morphotypes typical of monocotyledonous herbs in Zingiberales, most likely related to Costus or Canna , implying relatively moist habitats ( Supplementary Methods ). These zingiberaleans may have occupied small forest gaps along with open-habitat grasses but, overall, the combination of zingiberaleans and abundant, moisture-loving palms and closed-habitat grasses strongly indicates a landscape dominated by subtropical forest vegetation. If partially open vegetation, where wind transport would have been important (for example, grass–forest mosaics) was present, it should be reflected in more regionally mixed phytolith assemblages as substantial, albeit potentially variable grass abundances [15] . A small vegetation alteration occurred by ∼ 35 Myr ago, over 1 Myr before the Eocene–Oligocene global cooling event ( Fig. 3 ). Although palm phytoliths still dominate late Eocene-early Oligocene assemblages, zingiberalean forms disappear and grass short-cell abundances decrease. These assemblages appear to reflect forest communities with abundant palms in which grasses were scarcer than in the middle Eocene. We observe no vegetation change across the Eocene–Oligocene transition (EOT), in parallel with invariant terrestrial oxygen isotopic data ( Fig. 1 ) [19] . Early Miocene vegetation structure Vegetation composition shifts in the early Miocene. Grasses constitute significantly more of the vegetation overall, with grass short-cell abundances ranging from 0 to 25%. Morphotypes typical of the Pooideae (for example, stipoids) and PACMAD (for example, panicoids) clades dominate grass short-cell assemblages, whereas typical late Eocene closed-habitat grass and danthonioid?/bambusoid? forms are absent. In addition, palm phytoliths become less abundant. Despite more frequent grass phytoliths in some assemblages, short cell abundance falls below expectations for grass-dominated communities (>35–40% but more typically >>50%) (see Methods). Rather, Miocene assemblages continue to indicate forest vegetation, but with some more open areas where open-habitat grasses could thrive. These open microhabitats could potentially reflect spatially variable vegetation, for example, areas where water availability or disturbance regime favoured weedy open-habitat grasses over trees (for example, stream or lakes margins with intermittent sediment deposition, forest gaps). Alternatively, they could reflect temporal variation in seasonality, aridity or disturbance regime, allowing grasses to expand. Preliminary analysis indicates that short cell abundances are not higher in assemblages associated with tuffaceous sediment ( Supplementary Fig. S2 ), implying that grasses were not favoured after ash fall disturbance. Overall, the record of Eocene–Miocene vegetation at Gran Barranca demonstrates that the earliest grass-dominated habitats developed sometime after 18.5 Myr ago. This interpretation contrasts with previous phytolith-based reconstructions of the lower Sarmiento Formation that indicate that grassland vegetation was established by 40 Myr ago [10] , specifically at the level of the prominent Simpson’s Y ash. Multiple samples along and across this ash reveal spatial differences in palm abundance between the western and eastern part of the outcrop, but show consistently very low grass abundances ( Fig. 3 ). Both paleobotanical data and some fauna-based proxies further strongly suggest that these habitats were closed. The high frequency in phytolith assemblages of palms, which today are most abundant and diverse in humid forests and wetlands [20] , [21] , combined with the presence of zingiberaleans and/or closed-habitat grasses evident in phytolith assemblages until at least the early Oligocene indicates a landscape dominated by humid forest vegetation; similarly, the taxa that dominate macro- and palynofloras suggest closed forests growing under wet climates until at least the late Oligocene [13] , as do cenogram analysis of South American fossil faunas [22] . Local environments appear to have become patchier in the early Miocene ( Fig. 3 ) [13] , and it is worth noting that many herbivore lineages show significant increases in hypsodonty during this time ( Fig. 1 ). On the basis of these data, we reject the hypotheses that Earth’s first grass-dominated ecosystems appeared in Patagonia and that the early evolution of hypsodonty in southern South America was driven by the spread of grasslands. This differs sharply from the pattern seen on other continents where phytoliths directly associated with faunas have been analysed. In both central North America and the eastern Mediterranean, grass-dominated habitats preceded presumed grazers by several million years ( Fig. 4 ) [6] , [7] , indicating that, although delayed, hypsodonty plausibly evolved in response to the emergence of open, grass-dominated habitats, in accordance with traditional views [3] . Our results from Gran Barranca call this dogma into question, showing that grass dominance and openness of vegetation are not necessary pre-conditions for favouring high-crowned dentition. A different set of factors must be considered to explain the evolution of this trait. 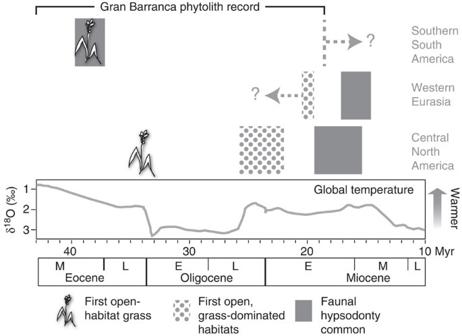Figure 4: Grassland ecosystem assembly in the Americas and western Eurasia. The timing of the appearance of open-habitat grasses and spread of grass-dominated habitats is based primarily on phytolith assemblage data and therefore limited to continents with detailed phytolith records. Width of grey/dotted boxes reflects age uncertainty. Global temperatures are based on stable oxygen isotope records from benthic foraminifera. References inSupplementary Information. Figure 4: Grassland ecosystem assembly in the Americas and western Eurasia. The timing of the appearance of open-habitat grasses and spread of grass-dominated habitats is based primarily on phytolith assemblage data and therefore limited to continents with detailed phytolith records. Width of grey/dotted boxes reflects age uncertainty. Global temperatures are based on stable oxygen isotope records from benthic foraminifera. References in Supplementary Information . Full size image What are these factors? In principle hypsodont forms could have migrated into Patagonia from other regions with different environmental stressors, but Patagonian mammals are always more hypsodont than coeval faunas across South America, and phylogenetic analyses fail to reveal sister taxa with higher-crowned teeth in older deposits elsewhere ( Supplementary Methods ). Instead, we favour consumption of abrasive materials unrelated to grasses, such as other silica-accumulating plants (for example, palms) or dietary grit. In particular, we note an abundance of ash in the Sarmiento Formation and location downwind of active Andean and intracontinental volcanoes. In addition to arc volcanism to the west in the Andean Volcanic Province, quasi-continuous back-arc volcanism occurred proximally to Gran Barranca from the early Eocene to Quaternary [23] , [24] . We hypothesize that continual replenishment and exposure of abrasive ash, and ash-rich soils, through explosive eruptions and surface processes could have provided selective pressures favouring the evolution of hypsodonty [25] , [26] . It is beyond the scope of this paper to collect the data necessary to test these alternative hypotheses, but we make the following observations. First, a body of work has shown that hypsodonty in modern ungulates correlates not just with diet, but with habitat openness, precipitation and feeding height, regardless of grass abundance [27] , [28] , [29] ; thus, there is current utility of high-crowned teeth in environments where abundant abrasives, such as soil particles or volcanic ash, are ingested alongside plant matter. In particular, a recent study implies that fine-grained volcanic ash abrades teeth without resulting in the wear patterns associated with ingestion of coarser grit [27] . Second, although high levels of ingested grit are typically associated with open, arid ecosystems, large mesodont–hypsodont herbivores do exist in some forest or woodland habitats today ( Fig. 1 in [28] ): either due to in situ cheek–tooth evolution or evolution elsewhere and subsequent immigration. This pattern can be compared with tooth wear studies in late Oligocene and Miocene hypsodont or hypselodont herbivores, suggesting that South American taxa with high-crowned cheek teeth were not limited to highly abrasive diets [30] , [31] . Third, volcanic ash deposited in tropical and temperate forests can lead to extreme tooth wear in animals (primates) feeding on dust-covered plants [32] . In a predominantly closed environment with frequent, distal ash deposition primarily affecting understory plants [33] , we suggest that feeding height or other types of niche partitioning (for example, according to plant toughness, affecting chewing effort [34] ) might lead to differential selective pressure for hypsodonty among herbivores, including marsupials [35] , rodents (post-Eocene) [36] and xenarthrans [37] . Unlike in younger strata [38] , Gran Barranca has yielded almost no cranial and post-cranial material that would allow refined reconstruction of functional morphology, and tooth wear data for members of lineages actively evolving hypsodonty in southern South America are not yet available; thus, this hypothesis remains untested. However, we note that some of the earliest lineages to acquire hypsodonty, archaeohyracids and interatheres ( Fig. 1 ) were small-bodied [26] , and may have been more sensitive to local factors of soil availability also in closed forests. Our data also challenge the long-standing notion that dense concentrations of dung beetle brood balls, starting at 40 Myr ago, necessarily reflect grassland ecosystems [11] . Several phytolith assemblages described herein come from horizons with dense concentrations of brood balls yet contain very little grass, consistent with previous phytolith analyses of dung beetle brood balls from southern South America [39] . At Gran Barranca and elsewhere, dung beetle brood balls are found in strata that have yielded primate fossils, typically viewed as clear indicators of forested habitats [40] . Furthermore, fossil evidence for Late Cretaceous dung beetles suggests that they thrived in forested, or at least grass-free ecosystems long before the evolution of large mammalian herbivores and savannah vegetation [41] . It can also be noted that the largest diversity of dung beetles in South and Central America today is found in tropical forests, not grasslands, and include taxa with a nesting behaviour that closely matches that reflected in Eocene–Miocene brood balls at Gran Barranca [42] , [43] . Other trace fossils described from the Gran Barranca section [44] are not specific to vegetation type and therefore do not contradict our environmental interpretation. The presence of members of the Pooideae and PACMAD clades at Gran Barranca from at least 38 Myr ago agrees with previous phytolith work in Patagonia [10] , [45] , adding to the body of evidence that open-habitat grasses diversified prior to the EOT [14] , [46] , [47] . Thus, the rise to ecological dominance of open-habitat grasses lagged taxonomic diversification by at least 20 million years in southern South America. This decoupling parallels the North American record [14] , suggesting that it reflects an evolutionary/ecological phenomenon rather than incomplete fossil records; similar patterns have been recorded in C 4 grasses [14] and several other organisms, such as early flowering plants and certain insect groups [48] , [49] . If true, the lag implies that different factors influenced pooid and PACMAD diversification versus ecological expansion [14] . What environmental (or other) changes allowed open-habitat grasses to become more abundant albeit not ecologically dominant in the Miocene of Gran Barranca? Tree cover in savannahs is determined mainly by annual rainfall and rainfall seasonality [50] , hence, the slight increase in open-habitat grasses over trees may suggest drier local climates. This scenario is consistent with the lower abundance of palms [20] . Alternatively, the increase in open-habitat grasses and, by inference, openness may relate to intensified disturbance in the form of ash fall, fire or herbivore pressure [51] . There is currently no charcoal evidence for fire regime changes, and declining dung beetle brood ball density during the earliest Miocene [11] suggests that herbivore abundance did not increase [52] . The pattern of volcanic disturbance is poorly studied at Gran Barranca during the early Miocene, but remains a possible explanation. Taken together, our results challenge the notion that convergent evolution necessarily reflects similar sets of environmental conditions, as has often been assumed [2] , [3] , [4] , [5] . Although it is still likely that environmental abrasiveness was the ultimate trigger for the evolution of hypsodonty, caution is required when using this functional trait for habitat reconstruction. In the case of hypsodonty, the past is the key to the past. Hypsodonty index Hypsodonty indices (HI, Fig. 1 , Supplementary Table S1 ) were taken from published compilations and from measurements provided by generous colleagues (see Supplementary Table S1 ). The maximum HI value for a species was used for all occurrences of that species. HI for molars equals maximum tooth crown (enamel) height divided by maximum anteroposterior tooth length, normally at the occlusal surface. This measure can dramatically underestimate HI because unworn molars do not exist for many notoungulates. This is particularly problematic for notoungulates exhibiting ever-growing (eledont/euhypsodont/hypseledont) teeth starting at 24 Myr ago. Thus, average and maximum HI are likely increasingly underestimated in younger teeth. Fieldwork and geologic framework Ten profiles (Colhue-Huapi West, A1-3, MMZ, J, K, L, M and N) along the 7-km-long Gran Barranca escarpment were sampled at high resolution (typically every 0.5–1 vertical metre) to get maximally complete temporal coverage through the Sarmiento Formation, amounting to 438 samples; in addition samples were taken from nearby Vacan-aged deposits. All available lithologies were collected, focusing on paleosols. Certain, prominent ash layers (for example, Simpson’s Y tuff, Bed 10) were sampled at different profiles to get spatial coverage along the Gran Barranca outcrop. For stratigraphic and lithologic information for the 58 samples described herein, see Supplementary Table S2 . Age model for phytolith samples The age model for the phytolith assemblages is based on the improved chronostratigraphic framework provided by Dunn et al. [18] ( Supplementary Table S3 ), but our conclusions are not dependent upon it. Ages for phytolith samples were based on stratigraphic position between horizons of known age, as determined from 40 Ar/ 39 Ar 17 and 206 Pb/ 238 U 18 radioistopic dating, or magnetostratigraphic correlation [16] , [18] . These age estimates assume constant sedimentation rate between dated horizons except where thick tuff units occur. Samples within the tuff units, which can be as thick as 3 metres, are assigned the same age as the tuff. For most stratigraphic units, upper and lower age constraints were possible; however, units such as ‘El Nuevo’ beds and Rosado member lack bracketing ages ( Supplementary Table S3 ). For these units, ages for the phytolith samples were estimated based on stratigraphic order. The age of ‘El Nuevo’ beds is uncertain, but the mammalian fossil assemblage contained within this 10-m thick unit appears evolutionarily younger than Barrancan faunas from the Gran Barranca member and older than Mustersan faunas from the Rosado member [8] . Therefore, we estimate ages for the phytolith samples in this unit to be younger than the top of the Gran Barranca member, and slightly older than the Rosado member between 38.05 and 38.04 Myr ago. The Rosado member ( ∼ 10-m thick) has a dated tuff, the Rosado Tuff (<38.03 Myr ago) at the top of the unit, but the base is of unknown age. We estimate that phytolith samples from this unit are 38.03–38.02 Myr ago based on their stratigraphic occurrence. An upper age for the lowermost Upper Puesto Almendra (UPA) in Profile A-2 (8-m thick) is also unknown. The base of the UPA is dated by the La Cantera Tuff (≤30.77 Myr ago) [18] , and the upper part occurs below a basalt flow dated at 27.76±0.08 Myr ago [17] . The basalt flow forms an unconformable surface but provides a maximum age for the top of the unit. The sedimentology of the unit suggests rapid deposition of tuffaceous materials in a paleochannel. Hence, we estimate UPA phytolith samples to be roughly the same age as the La Cantera Tuff. Two phytolith samples from Profile MMZ (UWBM 18456, UWBM 18457) were collected from a zone (6-m thick) of uncertain stratigraphy and age between the Lower and Upper Puesto Almendra members, specifically above a disconformity atop the Kay Tuff, but below the basalt flows of the UPA. The lithology of the unit is not distinctive, but the phytolith composition closely resembles samples of the Vera Member, which occurs farther east between Lower and Upper Puesto Almendra members. Therefore, we assign these samples to the Vera member. Phytolith extraction and classification Phytoliths were extracted from sediment using standard methods, in which 2–250 μm phytoliths are analysed together to avoid size-bias [53] . Slides are reposited in the Burke Museum of Natural History and Culture. Preservational state of phytoliths were assessed following Strömberg [7] ( Supplementary Table S4 ). Circa 140 samples were processed, all of which yielded biosilica of mainly fair to very good preservation. Of these, we analysed 58 assemblages, distributed throughout the Sarmiento Formation ( Supplementary Table S2 ). Scanning of remaining extracted assemblages revealed vegetation patterns fully consistent with that presented in Fig. 3 . Phytoliths were counted under a compound microscope at 1,000 × magnification using oil immersion, as lower magnification prevents recognition of small, but diagnostic, morphotypes (for example, grass silica short cells (GSSC)) [53] . The three-dimensionally complex GSSC (‘short cells’ in the text) were counted in immersion oil slides to allow rotation; GSSC and non-GSSC were subsequently counted in fixed slides. In 57 phytolith assemblages, over 200 diagnostic phytoliths (classes FI and GSSC in Supplementary Tables S4 and S5 and below) were typically counted to produce statistically reliable results [54] . Due to insufficient preservation, only a semi-quantitative assessment was made for assemblage UWBM no. PB18420 from the basal Sarmiento Formation at Gran Barranca ( Supplementary Table S4 ). Phytoliths were classified according to Strömberg [7] , [14] , using literature and a reference collection of phytoliths from modern plants (1,000 samples from >500 taxa of vascular plants) ( Supplementary Table S5 ). Some of our morphotypes correspond to morphotypes in the system used in previous studies of the Cenozoic of Patagonia [10] , [45] , initially devised by Bertoldi de Pomar [55] and expanded by subsequent workers [10] . However, our system differs in being based on quantitative assessment of distribution of morphotypes among plant taxa [56] . Diagnostic phytoliths are in classes PALM, ZINGI, other FI, CH TOT, POOID-D, POOID-ND, PAN, CHLOR, PACMAD general, OTGH and AQ ( Supplementary Tables S4 and S5 ), although note that AQ is not included in vegetation analysis ( [14] ). In addition, a set of tall bilobates and polylobates with faceted, slightly irregular tops were grouped under Danthonioideae?/Bambusoideae? (see Supplementary Methods ). For the quantitative analysis, they were included as PACMAD general, but their abundance in grass communities was also recorded semi-quantitatively ( Supplementary Table S4 ). Classes NDG and NDO are considered non-diagnostic and therefore excluded from vegetation analysis [7] . This omission differs from previous reconstructions of vegetation change in the Eocene–Miocene of Patagonia, Argentina [9] , [10] , [45] . Excluding, for example, elongate sinuous long cells, acicular hair cells and bulliforms from the sum of grass phytoliths reduces the inferred abundance of grasses relative to FIs, but does not fully explain the difference between our interpretation and that of previous authors [39] . Analysis of vegetation and habitat type We reconstructed vegetation type (grassland versus forest) by comparing (1) types and relative abundances of different FI phytoliths (PALM+ZINGI+other FI=FI) and diagnostic grass phytoliths (GSSC) and (2) the relative abundance of GSSC typical of grasses with preference for closed versus open habitats [7] , [14] ( Supplementary Table S4 ). Only broad patterns of relative change in vegetation structure are considered herein because of uncertainties introduced by the many factors that affect phytolith assemblage composition in different ecosystems [14] , [53] . However, in general, soil phytolith studies show that the abundance of grass phytoliths faithfully reflects the relative abundance of grasses in many modern ecosystems [15] , [53] —although note that authors disagree on what phytolith morphotypes should indicate grass cover (compare, for example, [57] [14] and 14). For example, applying the methods used herein to two large, modern phytolith data sets from West Africa [57] , [58] shows that grass-dominated vegetation (densely tree-covered savannah to open grasslands, including short grass steppe with shrubs) produces assemblages with, on average, 16.4% FI forms (of a sum of FI+GSSC), with maximum values in assemblages from dense tree/shrub savannah (53–64%) and short grass steppe with shrubs (11–58%) (data not shown). This suggests that grass-dominated habitats will typically produce phytolith assemblages with at least ∼ 35–40% GSSC, with assemblages from more open savannahs usually >>50% GSSC. Note that phytolith analysis reconstructs vegetation structure most accurately in tropical–subtropical regions whereas in some temperate ecosystems, FI phytoliths are underrepresented [53] . We inferred microhabitat and proximity to water using phytoliths typical of wetland plants (AQ), semi-quantitative abundance estimates of diatoms, sponge spicules and chrysophyte cysts, and sedimentology ( Supplementary Tables S2, S4 and S5 ; [59] ). We did not distinguish morphotypes typical of the Podostemaceae [10] , as these are also produced by FI taxa. Thus, a small subset of FI phytoliths may derive from this tropical–subtropical aquatic riverweed family. However, because most samples likely derive from soils distal to rivers, this potential, slight bias in favour of FI taxa would affect very few samples. Grass phytolith assemblage composition was assessed by examining the contribution of GSSC typical of (a) closed-habitat versus open-habitat grasses (CH TOT versus remaining GSSC classes) and (b) pooid versus PACMAD open-habitat grasses (POOID-D+POOID-ND versus PAN+CHLOR+PACMAD general). Because of the low GSSC frequencies in all samples, confidence intervals (not calculated) are likely to be wide [54] ; hence interpretation of grass community composition are semi-quantitative at this point. For Fig. 3 , we excluded non-diagnostic, unknown and unidentifiable GSSC (OTHG; on average 28% of GSSCs), and scaled diagnostic GSSC (minus OTHG) relative abundances to the total GSSC count. It is unlikely that this omission significantly skews our interpretation of GSSC assemblage composition [60] . How to cite this article: Strömberg, C.A.E. et al. Decoupling the spread of grasslands from the evolution of grazer-type herbivores in South America. Nat. Commun. 4:1478 doi: 10.1038/ncomms2508 (2013).